Multiple states in highly turbulent Taylor–Couette flow The ubiquity of turbulent flows in nature and technology makes it of utmost importance to fundamentally understand turbulence. Kolmogorov’s 1941 paradigm suggests that for strongly turbulent flows with many degrees of freedom and large fluctuations, there would only be one turbulent state as the large fluctuations would explore the entire higher dimensional phase space. Here we report the first conclusive evidence of multiple turbulent states for large Reynolds number, Re (10 6 ) (Taylor number Ta (10 12 )) Taylor–Couette flow in the regime of ultimate turbulence, by probing the phase space spanned by the rotation rates of the inner and outer cylinder. The manifestation of multiple turbulent states is exemplified by providing combined global torque- and local-velocity measurements. This result verifies the notion that bifurcations can occur in high-dimensional flows (that is, very large Re) and questions Kolmogorov’s paradigm. For macroscopic flows of water or air the Reynolds number is much larger than unity; the standard type of flow is therefore turbulent. A typical Reynolds number for a person walking is . For large airplanes the Reynolds number is , for atmospheric currents it is , and for ocean currents it is . Reynolds numbers are even larger for astrophysical problems [1] . It is not possible to achieve these large Reynolds numbers in a lab-environment nor is it accessible by direct-numerical simulations (DNS). To extrapolate data from to the scales of our atmosphere or the ocean we must bridge 4–5 decades in Reynolds number, and even more for astrophysical applications [2] . While scaling laws that can predict the rough magnitude of these flows exist, they are rendered impractical if there is a flow-transition from a turbulent state at lower Re to another turbulent state at higher Re, or if multiple turbulent states can coexist at the same Re. To extrapolate to large scales we need to know whether there are transitions and whether multiple states can coexist in high-Reynolds number flows. As an answer to this question, Kolmogorov’s more than 70-year-old paradigm states that for large Reynolds numbers, flows would become ‘featureless’ due to the fact that the highly dimensional phase space is explored in its entirety owing to the large fluctuations of said flows [3] , [4] . For Rayleigh–Bénard (RB) convection at low Rayleigh number (laminar-type boundary layers, Ra<10 14 ), continuous switching between two different roll states, with different heat transfer properties, was found [5] , [6] , [7] . In this case, the turbulent fluctuations were large enough to overcome trapping in one turbulent state. In the case of high Rayleigh number (turbulent boundary layers), no multiple states have been observed in a single setup; only when the boundary conditions were changed one could trigger a transition to a different state [8] , [9] . For von Kármán flow multiple turbulent states were found when driving it with impellors with curved blades [10] , [11] , [12] . These studies revealed the spontaneous symmetry-breaking and turbulent bifurcations in highly turbulent von Kármán flow up to Re=10 6 . In spherical-Couette flow Zimmerman et al . [13] observed spontaneous switching between two turbulent states at fixed rotation rates. The presence of coherent structures at high Reynolds numbers in closed systems suggests that Kolmogorov’s hypothesis [3] , [4] is incomplete [10] , [11] , [12] , [13] and might need revisiting to apply it to these flow systems. For Taylor–Couette (TC) multiple states are only observed for low Re (see for example, ref. 14 )—the so-called classical regime, where the bulk is laminar or turbulent but the boundary layers are still of laminar type. Around Re~\n10 4 (refs 15 , 16 ) the system transitions into the ultimate state [9] , [17] , [18] , in which the boundary layers are also turbulent [19] , and where new scaling laws of the response parameters set in [15] , [20] , [21] , [22] , [23] , [24] , [25] , [26] . Historically, this ultimate regime was defined based on the scaling properties of the flow [17] . Consequently, it does not necessarily exclude the existence of multiple turbulent states. To correctly extrapolate to much higher Re it is crucial to know the characteristics of the turbulent state and the existence of other such states. In ref. 27 it was shown that for increasing Re the waves on top of the Taylor vortices become increasingly complex until only turbulent Taylor vortices are left. Lewis et al . [28] came to the same conclusion by plotting the velocity power spectra for increasing Re up to 5 × 10 5 , and observed that the peaks gradually decrease in amplitude. They noted that turbulent Taylor vortices remained. On the other hand, the findings of Lathrop et al . [18] suggest that the Taylor vortices are not present for Reynolds numbers beyond 1.2 × 10 5 . Here we demonstrate that roll structures remain for TC flow even in the ultimate regime up to at least and show that multiple states are even possible far beyond the transition into this ultimate regime. System parameters For TC flow [15] , [21] , [22] , [23] , [24] , [25] , [26] and using the analogy of TC flow with RB convection [29] it was found that the Taylor number is a very well suited parameter to describe the driving of the system, see also the Methods section [30] . Here ω i , o =2π f i , o are the angular rotation rates and ν the kinematic viscosity. The response of the system is the torque required to sustain constant angular velocity or a ‘Nusselt’ number [30] , Nu ω = τ / τ lam , which is the angular velocity flux nondimensionalised with the flux of the laminar, nonvortical, flow. This Nusselt number scales approximately as Nu ω ∝ Ta 0.38 (refs 21 , 22 ) around Ta=10 12 , which is interpreted as Nu ω ∝ Ta 1/2 Log—corrections [9] , [17] . We now find with our new sensor with improved accuracy that the exponent is closer to 0.40 (results not shown), which is still consistent with the aforementioned interpretation. The Twente Turbulent TC facility (T 3 C) [31] was used for the experiments, see Fig. 1 and the Methods section for more details. 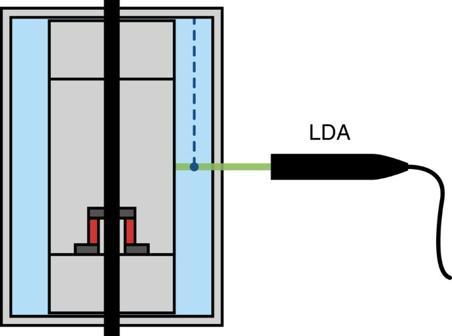Figure 1: Experimental apparatus. Schematic of the cross section of the T3C (ref.31): the apparatus has been outfitted with a new co-axial torque transducer (shown in red), see the Methods section. The azimuthal velocity is probed at the middle of the gap and in the top half of the apparatus using laser Doppler anemometry (LDA). Figure 1: Experimental apparatus. Schematic of the cross section of the T 3 C (ref. 31 ): the apparatus has been outfitted with a new co-axial torque transducer (shown in red), see the Methods section. The azimuthal velocity is probed at the middle of the gap and in the top half of the apparatus using laser Doppler anemometry (LDA). Full size image Explored phase space First we follow trajectory I and V shown in the parameter space of Fig. 2 , which have a characteristic that f i – f o =8 Hz (except for the initial and the final part) and is equivalent to Ta≈10 12 or . While traversing the trajectory we continuously measure the torque, scanning over a in one experiment. This is in contrast to experiments that were performed before, where the torque was measured by performing separate ramps of constant a =− f o / f i [18] , [21] , [22] , [23] , [26] . We slowly follow a trajectory in phase space, such as to be in a statistically quasi-steady state the entire time [21] . The temperature variation within the system is 0.04 K, the variation during each measurement is 0.3 K, and the mean temperature for each run is between 19°C and 24°C. The Taylor number depends on viscosity and thus temperature; we therefore remove the main temperature dependence by compensating the Nusselt number with Ta 0.4 , because Nu ω ∝ Ta 0.4 in the present parameter regime. This approach has been followed before, see for example refs 21 , 22 . 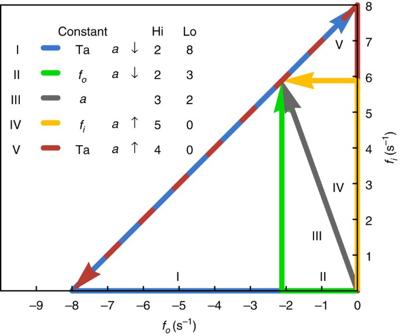Figure 2: Phase space of the trajectories I–V. The arrows indicate the direction in which the phase space is probed. The legend shows which parameter is kept constant, whether the parametera=−fo/fiis going down (a↓) or up (a↑), and the number of times it went to a high (Hi) or a low (Lo) state. All trajectories go through (or end at)fi=5.882 Hz andfo=−2.118 Hz (a=0.36, and Ta≈1012or Re≈106). Also, see the supplementary movie 1. Figure 2: Phase space of the trajectories I–V. The arrows indicate the direction in which the phase space is probed. The legend shows which parameter is kept constant, whether the parameter a =− f o / f i is going down ( a ↓) or up ( a ↑), and the number of times it went to a high (Hi) or a low (Lo) state. All trajectories go through (or end at) f i =5.882 Hz and f o =−2.118 Hz ( a =0.36, and Ta≈10 12 or Re≈10 6 ). Also, see the supplementary movie 1. Full size image Global torque and local velocity As can be seen in Fig. 3 , for increasing a (red shades, trajectory V), the torque is continuous and shows a peak around a =0.36, as found before [21] , [22] , [23] , [26] . For trajectory I the torque is found to be the same as trajectory V for a <0.17 and a >0.51, however for 0.17< a <0.51 the torque is found to be different. For decreasing a the system is able to enter another state around a =0.51, which is characterized by a lower torque (from here on called ‘low state’), around a =0.17 the system sharply jumps back to a higher torque state (‘high state’), see also the close up view in Fig. 4 . We have repeated these experiments to see how sharp this transition is, and to see in which state the system is, see Fig. 2 . For trajectory V we observe that it always goes into the high state, while for the reverse trajectory I the system goes to the low state (for 0.17< a <0.51) with a high probability (8 out of 10). 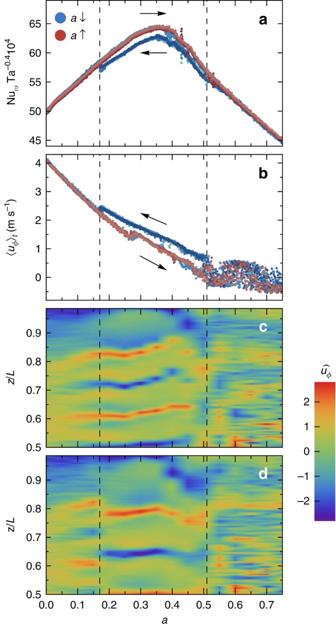Figure 3: Global torque and local velocity at different rotation ratios. (a) Compensated Nuωas a function ofa. Experiments following trajectories I and V are colored in blue and red, respectively. Experiments following trajectory I either go into a high or a low state for 0.17<a<0.51, while experiments of trajectory V are always in the high state. The stability of the two different turbulent states is clearly revealed. (b) Azimuthal velocity measured atr=(ri+ro)/2 andz/L=0.5 as a function ofafor trajectories I and V. Same colors as ina. For the local velocity we also see that the system bifurcates when following trajectory I arounda=0.51, either choosing the high or low state for 0.17<a<0.51. (c) and (d) show axial scans of the standardized angular velocity for varyingafollowing trajectories I and V, respectively. We see the presence of four rolls in the top half of the system inc, while indonly three rolls are present for 0.17<a<0.51. Fora<0.17 anda>0.51 the system is in the same state, regardless of the trajectory followed in phase space., where σais the standard deviation ofuφfor eachaand <>xstands for averaging over x. The torque of trajectory V is 2.5% larger than for trajectory I ata=0.36. Figure 3: Global torque and local velocity at different rotation ratios. ( a ) Compensated Nu ω as a function of a . Experiments following trajectories I and V are colored in blue and red, respectively. Experiments following trajectory I either go into a high or a low state for 0.17< a <0.51, while experiments of trajectory V are always in the high state. The stability of the two different turbulent states is clearly revealed. ( b ) Azimuthal velocity measured at r =( r i + r o )/2 and z / L =0.5 as a function of a for trajectories I and V. Same colors as in a . For the local velocity we also see that the system bifurcates when following trajectory I around a =0.51, either choosing the high or low state for 0.17< a <0.51. ( c ) and ( d ) show axial scans of the standardized angular velocity for varying a following trajectories I and V, respectively. We see the presence of four rolls in the top half of the system in c , while in d only three rolls are present for 0.17< a <0.51. For a <0.17 and a >0.51 the system is in the same state, regardless of the trajectory followed in phase space. , where σ a is the standard deviation of u φ for each a and <> x stands for averaging over x. The torque of trajectory V is 2.5% larger than for trajectory I at a =0.36. 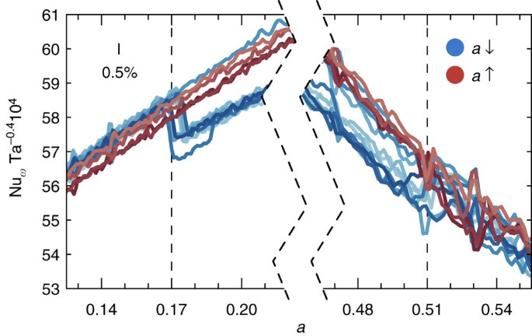Figure 4: Close up view ofFig. 3a. The trajectories I (a↓) that are in the low state sharply transition to the high state arounda=0.17. Trajectories I start to transition arounda=0.51, though the process seems more gradual, and sometimes stay in the high state. Trajectories V (a↑) never transition and are always in the high state. The error bar, shown in the top-left of the figure, is based on the accuracy of the torque sensor in the system. Full size image Figure 4: Close up view of Fig. 3a . The trajectories I ( a ↓) that are in the low state sharply transition to the high state around a =0.17. Trajectories I start to transition around a =0.51, though the process seems more gradual, and sometimes stay in the high state. Trajectories V ( a ↑) never transition and are always in the high state. The error bar, shown in the top-left of the figure, is based on the accuracy of the torque sensor in the system. Full size image To verify that the high- and low-torque states originate from two different physical states, we measure the azimuthal velocity at half-height z = L /2 and center of the gap r =( r i + r o )/2, while the system is let to move along trajectories I and V in phase space, see Fig. 3b . As in Fig. 3a , it is found that the local velocity inside the system bifurcates and that the two states are possible. The presence of multiple states in a local measurement (azimuthal velocity) and at the same time a global measurement (torque) provides convincing evidence that the system can indeed be in different turbulent states, despite the very high Taylor number of (ultimate regime). Flow structure To further characterize the turbulent state of the system, we perform axial scans of the azimuthal velocity in the top half of our apparatus for several a for both the high and the low state, see Fig. 3c,d . For each a the azimuthal velocity is standardized (zero mean, unit s.d.) and color-coded. Figure 3c shows the local velocity for the high state (trajectory V), and shows the presence of five large minima/maxima for a ≤0.45; a clear characteristic of four turbulent Taylor vortices. For a ⩾ 0.5 the state of the system is less clear, and the system appears to jump between states (without a well-defined a dependence), as seen in the local velocity in Fig. 3b . This behavior looks similar to what was found in RB convection in the classical turbulent regime [7] . However, the mechanism is different owing to the shorter turnover time scale of the TC system, and the presence of the additional control parameter a in TC, with which we can control the transition. Furthermore, the observed transition is different from ref. 13 where spontaneous switching back and forth between two states was found, based on global and local measurements. Figure 3d shows the same switching behavior as the high state of Fig. 3c for a outside [0.17,0.51]. For 0.17< a <0.51 it is found that the azimuthal velocity has four large minima/maxima, which is the signature of three turbulent Taylor vortices (in the top half of the system). In addition, we provide, for selected a , the angular velocity profiles as lines in Fig. 5 . The angular velocity profiles for trajectories I and V are identical (within experimental and statistical error) for a outside [0.17,0.51]. For a ε[0.17, 0.51] the profiles are different and show distinguishing features of three or four rolls (six and eight rolls in the entire setup), see also the schematics on the right of Fig. 5 . At the boundary of the last (top) roll and the penultimate roll, high-velocity fluid from the inner cylinder is advected towards the middle, increasing the velocity at the center of the gap. Similarly, at the boundary of the penultimate and the antepenultimate roll the low-velocity fluid from the outer cylinder is advected inwards, decreasing the velocity at the center of the gap. The corresponding average aspect ratio of the vortices is 1.96 (three rolls) and 1.46 (four rolls), which is consistent with previous studies (see for example, Figs 2 and 5 in ref. 32 ). Close inspection of Figs 3c and 5a shows that the roll around z / L =0.5 slightly drifts upwards for 0.3< a <0.45 (compared with a <0.3), which could be a signature of symmetry breaking; the top half of the system behaves slightly different from the bottom half. This is an explanation of the anomaly in the local-angular velocity for trajectory V around a ≈0.3. Such symmetry-breaking behavior has also been found in von Kármán flow [33] . 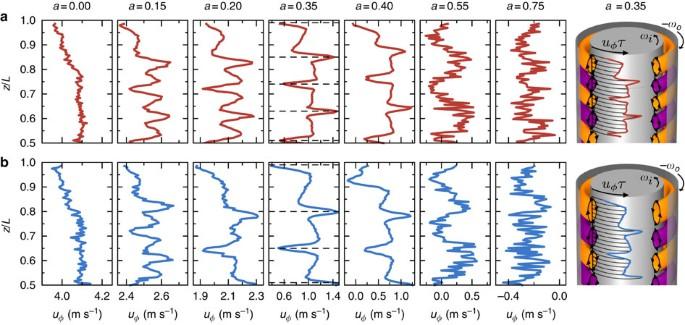Figure 5: Flow structures at different rotation ratios. Azimuthal velocity as a function of heightz/Lfor variousa. Subset of the data shown inFig. 3c,d. (a) Profiles following trajectory V. (b) Profiles following trajectory I. Foraε{0.00,0.15,0.55,0.75} the velocity profiles are the same for both trajectories. For intermediate values (aε{0.20,0.35,0.40}) the profiles are different; trajectory V (red) shows the emergence of four rolls in the top half of the system, while trajectory I (blue) shows only three rolls in the top half of the system. For the case of maximum torque (a=0.35), dashed lines are drawn to indicate the boundaries between the rolls. Fora=0.15 the system shows the high state (with four rolls in the top half). This structure seems to fade once the system is pushed towardsa=0, see alsoFig. 3c,d. On the right we show a schematical overview of the rolls and the angular velocity profile fora=0.35 in 3D,τ=0.2 s. Figure 5: Flow structures at different rotation ratios. Azimuthal velocity as a function of height z / L for various a . Subset of the data shown in Fig. 3c,d . ( a ) Profiles following trajectory V. ( b ) Profiles following trajectory I. For a ε{0.00,0.15,0.55,0.75} the velocity profiles are the same for both trajectories. For intermediate values ( a ε{0.20,0.35,0.40}) the profiles are different; trajectory V (red) shows the emergence of four rolls in the top half of the system, while trajectory I (blue) shows only three rolls in the top half of the system. For the case of maximum torque ( a =0.35), dashed lines are drawn to indicate the boundaries between the rolls. For a =0.15 the system shows the high state (with four rolls in the top half). This structure seems to fade once the system is pushed towards a =0, see also Fig. 3c,d . On the right we show a schematical overview of the rolls and the angular velocity profile for a =0.35 in 3D, τ =0.2 s. Full size image From our findings of trajectory I and V (constant Ta) we find that the maximum torque is at a =0.36 ( f i =5.882 Hz, f o =−2.118 Hz). We now look at other trajectories reaching this maximum but keeping either f o , a or f i constant, see trajectories II–IV in Fig. 2 . For constant f o and constant a (trajectories II and III) the system was found to have the ability to go in either the high or the low state as well, see the legend of Fig. 2 . Like trajectory V, trajectory IV (constant f i ) was found to be characterized by a high state of the system. It seems that if a =0.36 is approached from below (trajectories IV and V) the flow does not bifurcate. However, the system does bifurcate when a =0.36 is approached from the top, or if a is kept constant but the driving strength is increased. We have shown that TC flow displays flow structure even for a very high Taylor number of roughly 10 12 ( (10 6 )), which is beyond Reynolds numbers for which large-scale structures were believed to vanish in Kolmogorov’s picture. In addition, we found that the system is hysteretic and can be in multiple stable turbulent states for the same driving parameters. The multiple states are simultaneously measured globally and locally by performing torque and laser Doppler anemometry (LDA) measurements. It was found that multiple states can occur for rotation ratios 0.17< a <0.51. For 0≤ a <0.17 there is only a single-stable state, though we cannot exclude that other trajectories in phase space might trigger multiple states in this region. For a >0.51 the system does not posses a state with a clear roll structure. Presently, a theoretical understanding of the values a =0.17, a =0.51 and the sharp and smooth behaviour of the jumps around those a is lacking. Finally we note that the presented experiments, performed in the T 3 C facility, will be challenging to simulate in direct-numerical simulations in the foreseen future. Simulations of such high Ta are difficult, especially for . The present work highlights the importance of the coherent structures and their selectability in highly turbulent flows, which demand continued effort and investigation. The question of whether or not these structures survive for even larger Reynolds numbers, remains open but is important for understanding the myriad of large-scale flows in nature. Experimental apparatus The T 3 C (ref. 31 ) has an inner cylinder with an outer radius of r i =200 mm, a transparent outer cylinder with inner radius r o =279 mm, and a height of L =927 mm, giving a radius ratio of η = r i / r o =0.716 and an aspect ratio of Γ = L /( r o – r i )=11.7. The top and bottom caps rotate along with the outer cylinder. The apparatus was filled with water and actively cooled to keep the temperature constant. Torque measurements The torque is measured on the middle section of the inner cylinder using a new co-axial torque transducer (Honeywell 2404-2K, maximum capacity of 225 Nm), with improved accuracy compared with our former load cell [21] . The middle section of the inner cylinder with height z / L =0.578 does not cover all the rolls, therefore the exact mean torque value over the entire inner cylinder could be different. It is, however, unlikely that this difference takes away the ‘jumping’ behavior mentioned before. Velocity measurements The azimuthal velocity is obtained by LDA, see Fig. 1 . The laser beams go through the outer cylinder and are focused in the middle of the gap, see Fig. 1 The water is seeded with 5 μm diameter polyamide tracer particles (Dantec) with a maximum Stokes number of St= τ p / η K =0.004 ≪ 1. Curvature effects of the outer cylinder to our LDA system are accounted for by numerically ray-tracing the LDA-beams [34] . How to cite this article: Huisman, S. G. et al . Multiple states in highly turbulent Taylor–Couette flow. Nat. Commun. 5:3820 doi: 10.1038/ncomms4820 (2014).